A large family of filled skutterudites stabilized by electron count The Zintl concept is important in solid-state chemistry to explain how some compounds that combine electropositive and main group elements can be stable at formulas that at their simplest level do not make any sense. The electronegative elements in such compounds form a polyatomic electron-accepting molecule inside the solid, a ‘polyanion’, that fills its available energy states with electrons from the electropositive elements to obey fundamental electron-counting rules. Here we use this concept to discover a large family of filled skutterudites based on the group 9 transition metals Co, Rh, and Ir, the alkali, alkaline-earth, and rare-earth elements, and Sb 4 polyanions. Forty-three new filled skutterudites are reported, with 63 compositional variations—results that can be extended to the synthesis of hundreds of additional new compounds. Many interesting electronic and magnetic properties can be expected in future studies of these new compounds. The chemical stability of simple ionic compounds can be explained by fundamental concepts through which an electropositive ion donates electrons to an electronegative ion and both achieve closed shell electron configurations. NaCl, with Na 1+ , configuration 2 s 2 2 p 6 , and Cl 1− , configuration 3 s 2 3 p 6 , is the canonical example. For many compounds, however, the electron-counting and stability rules are not as straightforward. The Zintl phases are a family of solid compounds typically made from electropositive metallic elements combined with non-metals or metalloids capable of forming polyanions [1] . The more electropositive elements donate their valence electrons to the more electronegative elements, and the electronegative elements form polyanions to accept the donated electrons. The bonding and architecture of the polyanions is understood in terms of the octet rule [2] , [3] , [4] . Due to the filled valence states of the polyanion array and the empty valence states of the electropositive electron donors, semiconducting behaviour is favoured for the resulting compounds. The binary skutterudites are one well known class of Zintl compounds, deriving from the archetypal mineral skutterudite, CoAs 3 (refs 4 , 5 ). They have the general formula BX 3 , where B is a transition metal element such as Fe, Co, Rh or Ir and X is a pnictogen such as P, As or Sb (see Fig. 1a ) [5] , [6] , [7] ; they typically crystallize in cubic space group Im (#204) with two B 4 X 12 formula units and two large empty cages per unit cell. The B ions are in the 8c (1/4, 1/4, 1/4) site and the X ions are in the 24g (0, y , z ) site with y ~0.15 and z ~0.35. Featured in the structure are distorted square X 4 Zintl polyanions that have a formal charge of 4−. Thus, the simple binary compounds have a semiconducting electron count for B elements from group 9; the B ions, Co, Rh and Ir, formally 3+, have the electron configuration nd 6 . In octahedral coordination and low spin, they thus have a filled t 2 g band and an empty e g band, with an energy gap between them. CoAs 3 , for example, can be understood as Co 3+ 4 (As 4 ) 4− 3 (refs 8 , 9 , 10 ). 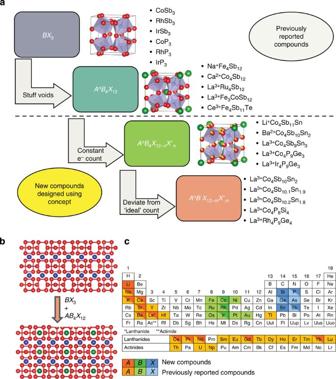Figure 1: Design of filled skutterudites using the Zintl concept and summary of current and previously reported stuffed skutterudites. (a) Flowchart for designing new skutterudites using the Zintl concept. (b) Structures ofBX3andAB4X12showing the covalently bonding regions (red atoms) separate from the ionic regions (blue and green atoms). The atoms in the two regions can be partially substituted for tuning of the electron concentration to change the electronic structure. (c) Periodic table of the elements highlighted to show the new stuffed skutterudites found in this work and those reported previously. Figure 1: Design of filled skutterudites using the Zintl concept and summary of current and previously reported stuffed skutterudites. ( a ) Flowchart for designing new skutterudites using the Zintl concept. ( b ) Structures of BX 3 and AB 4 X 12 showing the covalently bonding regions (red atoms) separate from the ionic regions (blue and green atoms). The atoms in the two regions can be partially substituted for tuning of the electron concentration to change the electronic structure. ( c ) Periodic table of the elements highlighted to show the new stuffed skutterudites found in this work and those reported previously. Full size image The empty cages within the binary skutterudite framework can be filled by up to one ion ( A ) per B 4 X 12 formula unit, leading to the ‘filled skutterudites’ of formula A y B 4 X 12 , where A =alkali, alkaline-earth, rare-earth, actinide or Tl (see Fig. 1b ) [11] , [12] , [13] . These are also in space group #204, with the A ions (in the ideal structures) in the 2a (0,0,0) site and the B and X ions as in the unfilled case. The known filled skutterudites are virtually all based on the group 8 metals Fe, Ru and Os. The A ion donates its charge to the B 4 X 12 framework. By judicious choice of constituents, complete filling of the cages ( y =1), a Zintl (electron precise) electron count, and thus semiconducting behaviour can be achieved. In addition to those with an electron-precise formula, some compounds such as LaRu 4 Sb 12 (with one electron in deficit of the Zintl count) are also known. A very small number of filled skutterudites based on Co, Ni and Pt have been reported (see Fig. 1c ) [14] , [15] , [16] , [17] , [18] , [19] , [20] , [21] , [22] , [23] , [24] , [25] , [26] , [27] , [28] , [29] , [30] , [31] , [32] , [33] , [34] , [35] , [36] , [37] , [38] , [39] , [40] , [41] , [42] , [43] , [44] , [45] , [46] . In addition to their chemical interest, skutterudites are of interest to a broad community of materials scientists and physicists due to their interesting physical properties. Because they make very good thermoelectrics [21] , [22] , [47] , host unusual metal–insulator transitions [23] , [24] , [25] , can be rare-earth magnets, heavy-fermion compounds [26] , [27] , [28] , [29] , [30] , non-Fermi liquids [31] , [32] , [33] , [34] , [35] , itinerant ferromagnets [36] , [37] , [38] and superconductors [27] , [39] , [40] , [41] , [42] , [43] , [44] , [45] , [46] , and have been proposed as topological insulators [48] , filled skutterudites are a very important class of non-molecular solids. Because the electronic and magnetic properties of solids depend critically on the actual atoms making up the compounds in addition to the compound’s electron count, expanding the filled skutterudites from primarily group 8 to group 9 metal-based compounds, as we have done in this study, affords the opportunity to observe many new physical properties. Here we report that an extremely large family of filled skutterudites based on the group 9 metals Co, Rh and Ir can be chemically stabilized if the electron count is stabilized by partial substitution on the X ion site to yield electron-precise formulas. These new filled skutterudites were designed by filling or partial filling the cages in the binary CoSb 3 , RhSb 3 and IrSb 3 frameworks with alkali (Li, Na and K), alkaline-earth metal (Ca, Sr and Ba) and rare-earth atoms (La, Ce, Pr, Nd, Gd and Yb), by compensating for the extra-positive charge of the filling ion by partial substitution of Sn on the Sb site or Si on the P site to yield electron-precise formulas, guided by the predictions of first principles electronic structure calculations. The pure antimonides and pure phosphides (with no Sb/Ns or P/Si mixing) are not stable, but we find that electron-precise formulas are not strictly required for compound stability in some cases. In addition to their synthesis, crystal structures and electronic structures, we briefly survey the magnetic properties of selected members of this large new family of compounds. Electronic structure and prediction The prototypical binary BX 3 skutterudites with B =Co, Rh and Ir are non-magnetic semiconductors with a Zintl electron count of 24 valence electrons per formula unit. (The 24 electron count rule per BX 3 unit for semiconducting behaviour also holds for a recently proposed non-Zintl view of the formal electron configuration of the constituent elements in skutterudites [49] .) Filled AB 4 X 12 skutterudites that have B in a d 6 low spin configuration and a p 6 X atom configuration are expected to be at electron precise, semiconducting, non-magnetic compounds when they have a valence electron count of 96 (4 × 24) per formula unit. The power of the Zintl concept is that these simple electron-counting rules enable the prediction of new thermodynamically stable compounds. A cobalt-based filled skutterudite compound can be stabilized, for example, by using Ba as an A 2+ ion and compensating for the added electrons by removing two electrons from the X ion site, and thus BaCo 4 Sb 10 Sn 2 should be stable, and an electron precise, non-magnetic semiconductor. In the same manner, the Rh and Ir compounds can be obtained as can the filled skutterudite semiconductors for any A ion. This simple electron count principle is confirmed by our ab initio calculations for several examples in this family, which are shown in Fig. 2a,c,e . The valence band consists of strongly hybridized metal d and pnictogen p states and is separated by a gap from the conduction band showing the expected semiconducting character. Our results for the current compounds are similar to those of ab initio calculations performed previously on other skutterudites [50] , [51] , [52] . Surprisingly, the electronic structure of the Rh variant calculated with the generalized gradient approximation (GGA) is semimetallic. Use of the Tran-Blaha Modified Becke-Johnson (MBJ) functional in the calculation [49] , which accounts for electronic correlations more effectively, on the other hand predicts the Rh variant to be a semiconductor. The results of the MBJ functional calculation are shown in Supplementary Fig. 1 . The calculated band structure of skutterudites around the Fermi level is very sensitive to changes in the lattice constants and internal parameters, as well as the chosen density functional theory (DFT) [48] , [53] . Since we are interested in the stability of the compounds, the qualitatively correct behaviour shown here is sufficient for our discussions [54] . 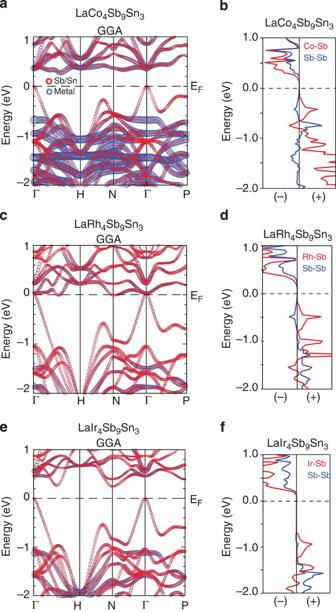Figure 2: Eelectronic structures of representative group 9 filled skutterudites. (a,c,e) Calculated electronic structures of the filled skutterudites LaCo4Sb9Sn3, LaRh4Sb9Sn3and LaIr4Sn9Sn3using the GGA functional. (b,d,f) Results of TB-LMTO-ASA (local density approximation)66,69electronic structure calculations on La[Co/Rh/Ir]4Sb12model compounds with La on 2a sites, Co/Rh/Ir on 8c sites and Sb/Sn on 24g sites.COHP curves between Co/Rh/Ir-Sb and Sb-Sb. Figure 2: Eelectronic structures of representative group 9 filled skutterudites. ( a , c , e ) Calculated electronic structures of the filled skutterudites LaCo 4 Sb 9 Sn 3 , LaRh 4 Sb 9 Sn 3 and LaIr 4 Sn 9 Sn 3 using the GGA functional. ( b , d , f ) Results of TB-LMTO-ASA (local density approximation) [66] , [69] electronic structure calculations on La[Co/Rh/Ir] 4 Sb 12 model compounds with La on 2a sites, Co/Rh/Ir on 8c sites and Sb/Sn on 24g sites.COHP curves between Co/Rh/Ir-Sb and Sb-Sb. Full size image The chemical concept behind the stability of these compounds is, furthermore, supported by crystal orbital Hamilton population (COHP) calculations using the tight-binding linear-muffin-tin-orbital (TB-LMTO) method, with the corresponding calculations shown in Fig. 2b,d,f . The COHP curves are used to indicate bonding and anti-bonding interactions. Here they show the presence of bonding interactions below the Fermi level in La[Co/Rh/Ir] 4 Sb 9 Sn 3 , while anti-bonding contributions are found above the Fermi level. This indicates that the filled skutterudite structure maximizes its bonding interactions at the electron count of 96 valence electrons per formula unit—the principle used here to synthesize the large new family reported. Structural characterization The compositions of the filled skutterudites was determined by standard solid-state phase equilibria methods, which, using the characterization of reaction products by powder X-ray diffraction (XRD), especially for the heavy elements in compounds such as these, is quite sensitive to the presence of impurities. In addition, the crystal structures of all 63 variants reported here were determined by quantitative fits to the powder diffraction patterns. 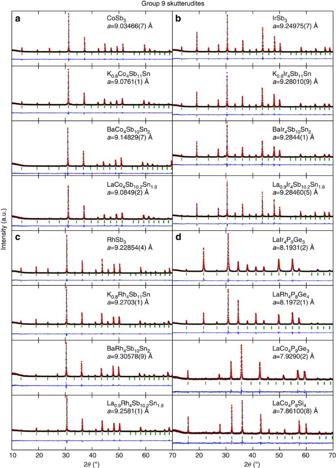Figure 3: Rietveld refinements for representative group 9 filled skutterudites. (a) CoSb3, K0.8Co4Sb11Sn, BaCo4Sb10Sn2and LaCo4Sb10.2Sn1.8. (b) RhSb3, K0.8Rh4Sb11Sn, BaRh4Sb10Sn2and La0.9Rh4Sb10.2Sn1.8. (c) IrSb3, K0.8Ir4Sb11Sn, BaIr4Sb10Sn2and LaIr4Sb10.2Sn1.8. (c) LaCo4P9Ge3, LaRh4P8Ge4, LaIr4P9Ge3and LaCo4P9Si3. Red points are observed data; black curves are the calculated pattern; green tics are expected peak positions; the lower blue curve is the difference between observed and calculated diffraction pattern. Refined structural parameters are found inTable 1. Figure 3 shows the powder XRD patterns for the quantitative Rietveld structure refinements for 12 examples of compounds the Co-series, Rh-series, Ir-series and P-series filled skutterudites. The agreement between the observed and calculated patterns in all cases is excellent; a selection of the structural refinements is shown in Table 1 with the remainder given in the Supplementary Information in Supplementary Table 1 . The cubic crystallographic cell parameters for all the compositions synthesized, determined by least squares fitting to 20 or more observed reflections in the powder XRD patterns using profile fits, are found in Table 2 . Figure 3: Rietveld refinements for representative group 9 filled skutterudites. ( a ) CoSb 3 , K 0.8 Co 4 Sb 11 Sn, BaCo 4 Sb 10 Sn 2 and LaCo 4 Sb 10.2 Sn 1.8 . ( b ) RhSb 3 , K 0.8 Rh 4 Sb 11 Sn, BaRh 4 Sb 10 Sn 2 and La 0.9 Rh 4 Sb 10.2 Sn 1.8 . ( c ) IrSb 3 , K 0.8 Ir 4 Sb 11 Sn, BaIr 4 Sb 10 Sn 2 and LaIr 4 Sb 10.2 Sn 1.8 . ( c ) LaCo 4 P 9 Ge 3 , LaRh 4 P 8 Ge 4 , LaIr 4 P 9 Ge 3 and LaCo 4 P 9 Si 3 . Red points are observed data; black curves are the calculated pattern; green tics are expected peak positions; the lower blue curve is the difference between observed and calculated diffraction pattern. Refined structural parameters are found in Table 1 . Full size image Table 1 Structural parameters for refined crystal structures of selected filled skutterudites and comparison to binary skutterudites. Full size table Table 2 Cubic cell parameters and selected physical properties of group 9-based filled skutterudites. Full size table Supplementary Figures 2–4 show the Rietveld refinements of the laboratory powder XRD data for the filled skutterudites made in this work. The ideal filled skutterudite structure is primarily found, with random Sb/Sn and P/Si mixing on the X ion site. For all the filled skutterudites based on P, and for the Sb-based variants based on Co, the A ions are found in the centres of the skutterudite cages (the 2a, (0,0,0) site), their ideal positons, as is frequently assumed for filled skutterudites in other chemical families. It is of interest, however, that for the compounds with the larger B ions, and consequently larger unit cells and X cages, we find that the A ions are sometime displaced from the centres of the cages, that is, off the ideal 2a site. This is found for the Ir compounds in particular. The qualitative evidence for this displacement is seen in comparing Fig. 3a to Fig. 3b,c ; it can be seen that the intensities of the low-angle diffraction peaks are suppressed by when the Co-skutterudites are filled, but that there is residual intensity seen in the Rh and Ir skutterudites. The three models evaluated to best model the observed diffraction peak intensities, rather than employing the ideal filled skutterudite structure, were: (a) refine the 2a site occupancy, (b) refine the 2a site atomic displacement parameter and (c) move the A atom off the ideal 2a site towards the surrounding X cage. Model (a) is not appropriate because the samples are single phase at the stoichiometry determined by phase equilibria studies; the formulas were further confirmed by energy dispersive X-ray spectroscopy. Model (b) provides an adequate fit, yielding excessively large atomic displacement parameters, implying that the A site ions are dynamically displaced from their ideal positions. The alternative model (c), where the A atom is randomly displaced to partially occupy sites along a <111> type direction to minimize the A-X distances in the cage, seems like the most physically realistic scenario and was the model used here to describe the rare-earth ion disorder. In a handful of cases, BaIr 4 Sb 10 Sn 2 and La 0.9 Ir 4 Sb 10.2 Sn 1.8 , for example, realistic off-centre A atom positions cannot sufficiently fully account for the observed intensities of the low-angle peaks, and thus it may be that a small fraction of the A ions are substituted on the B atom sites. Although the existence of 5 d Os and Pt rare-earth filled skutterudites been reported in the past [9] , [10] , [54] , [55] , few quantitative structure determinations have been reported. A model like (b), with anomalously large atomic displacement parameters for the lanthanides, has been used to describe the Ln site disorder for Os-based pyrochlores [56] . The very low thermal conductivity of the filled skutterudites based on group 8 elements has been attributed to the anharmonic thermal vibration of the A site ion ‘rattling’ in the skutterudite cage [47] , [57] , implying a tendency towards off-centre positioning of the A site ion in the cages in this family, in agreement with our structural refinements and those where the A site ion disorder is modelled by large thermal parameters. It is not yet known whether the A site disordered position model we observe here is a general feature of all larger filled skutterudites. Whether the disorder is static or dynamic or a combination of both, and whether there is any complex defect chemistry present in some of these compounds, would be of interest to study further by other structural characterization methods. The important structural features of the filled skutterudites studied here are presented in Fig. 4 . This figure shows the geometry of the A site and group 9 site polyhedra and the manner in which they share faces (leading to the strong anti-bonding interactions described above), the displacements of the A site ions from the cage centres and the X 4 squares. The lower part of the figure compares the X–X bond lengths within the slightly distorted X 4 antimonide and phosphide squares and the B–X bond lengths (all six are equivalent) for several representative members of the group 9 filled skutterudites. Neither the X 4 ‘squares’ nor the BX 6 octahedra are constrained by symmetry to be regular, and they are not, although they are all close to regular and the distortions are relatively small. Because the same electron count is nearly perfectly maintained for all the compounds studied quantitatively here, large bond-length differences in these critical structural components are not expected to occur. 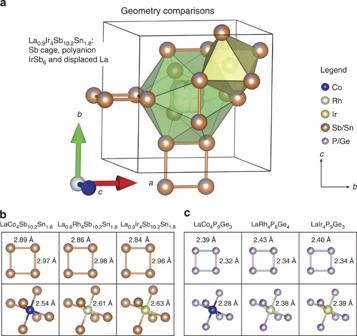Figure 4: Fragment of the filled skutterudite structure and comparisons of theX4square andBX6octahedron geometries for selected group 9 filled skutterudites. (a) Details of theAX12polyhedron, theBX6octahedron, theAsite displacement and theX4squares, and the manner in which they are related in the La0.9Ir4Sb10.2Sn1.8filled skutterudite. (b,c): Comparisons of theX4square andBX6octahedra geometries for selected filled group 9-based skutterudite compounds, from the current structure refinements. Figure 4: Fragment of the filled skutterudite structure and comparisons of the X 4 square and BX 6 octahedron geometries for selected group 9 filled skutterudites. ( a ) Details of the AX 12 polyhedron, the BX 6 octahedron, the A site displacement and the X 4 squares, and the manner in which they are related in the La 0.9 Ir 4 Sb 10.2 Sn 1.8 filled skutterudite. ( b , c ): Comparisons of the X 4 square and BX 6 octahedra geometries for selected filled group 9-based skutterudite compounds, from the current structure refinements. Full size image Magnetic properties Filled skutterudites based on rare-earth metals and group 8 transition elements show diverse and interesting rare-earth magnetism, and they have been widely studied (see, for example, refs 28 , 29 , 31 ). To generally survey the magnetic properties for our new filled group 9-based skutterudites, the magnetizations of all the rare-earth-based filled skutterudites were measured from 2 to 200 K with an applied magnetic field of μ 0 H =1 Tesla. The compounds are strongly paramagnetic as expected due to the rare-earth magnetism. We consider the analysis of several set of compounds in more detail as examples. 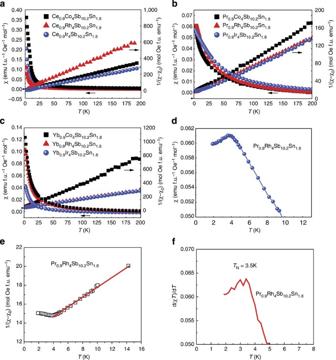Figure 5: Magnetic properties of selected group 9 filled skutterudites. (a) Ce0.9[Co/Rh/Ir]4Sb10.2Sn1.8; (b) Yb0.9[Co/Rh/Ir]4Sb10.2Sn1.8; and (c) Pr0.9[Co/Rh/Ir]4Sb10.2Sn1.8. (d) Enlarged low-temperature region of the magnetic susceptibility of Pr0.9Rh4Sb10.2Sn1.8. (e) Enlarged low-temperature region of the inverse susceptibility. (f) Enlarged low-temperature region of d(χT)/dT. Figure 5a–c shows in the main panel the inverse magnetic susceptibilities ( χ is defined as M / μ 0 H ) for the Ce 0.9 [Co/Rh/Ir] 4 Sb 10.2 Sn 1.8 , Yb 0.9 [Co/Rh/Ir] 4 Sb 10.2 Sn 1.8 and Pr 0.9 [Co/Rh/Ir] 4 Sb 10.2 Sn 1.8 samples. The temperature dependences of the inverse magnetic susceptibilities, corrected for χ 0 , are linear at high temperatures for all three compounds, indicating Curie Weiss behaviour. Fits to the susceptibilities were performed in the temperature range of 100–200 K, according to χ − χ 0 = C /( T − θ cw ), where C is the Curie constant, θ cw is the Weiss temperature and χ 0 is the temperature independent contribution to the susceptibility. From these fits, the effective magnetic moment ( P eff ) per Ln (Ln=La, Ce, Pr, Nd, Gd and Yb) ion was obtained by using P eff =(8 C ) 1/2 . The thus derived basic magnetic characteristics (that is, θ cw and P eff ) for all our new compounds containing magnetic rare earths are summarized in Table 2 . Fitting the magnetic susceptibility using the Curie Weiss law in the range 100–200 K, we obtain the effective moments for Pr 0.9 Co 4 Sb 10.2 Sn 1.8 , Pr 0.9 Rh 4 Sb 10.2 Sn 1.8 and Pr 0.9 Ir 4 Sb 10.2 Sn 1.8 of P eff =3.43, 3.66 and 3.66 μ B /Pr, respectively, close to the effective moment value expected for the free Pr 3+ -free ion ( P eff =3.58 μ B /Pr). In addition, the magnetic susceptibility data show a broad peak at around 3.5 K for Pr 0.9 Rh 4 Sb 10.2 Sn 1.8 ( Fig. 5d,e ), which implies the onset of antiferromagnetic ordering. To better estimate the Neel temperature, we follow standard procedure [58] , [59] and plot d( χT )/d T ( Fig. 5f ). The maximum of d( χT )/d T is observed at 3.5 K, which can be taken as T N . Similar fits were performed for all the rare-earth compounds synthesized. Figure 5: Magnetic properties of selected group 9 filled skutterudites. ( a ) Ce 0.9 [Co/Rh/Ir] 4 Sb 10.2 Sn 1.8 ; ( b ) Yb 0.9 [Co/Rh/Ir] 4 Sb 10.2 Sn 1.8 ; and ( c ) Pr 0.9 [Co/Rh/Ir] 4 Sb 10.2 Sn 1.8 . ( d ) Enlarged low-temperature region of the magnetic susceptibility of Pr 0.9 Rh 4 Sb 10.2 Sn 1.8 . ( e ) Enlarged low-temperature region of the inverse susceptibility. ( f ) Enlarged low-temperature region of d( χT )/d T . Full size image The effective moments for the Ce 0.9 [Co/Rh/Ir] 4 Sb 10.2 Sn 1.8 samples are in the range P eff =2.1–2.5 μ B /Ce, which are close to the expected free-ion Hund’s rule value of 2.54 μ B /Ce 3+ . These values are similar to the effective moment ( P eff =2.1–2.26 μ B /Ce) reported for the group 8 filled skutterudites CeRu 4 Sb 12 (ref. 32 ), but are different from those reported for CeFe 4 Sb 12 ( P eff =3.5–3.8 μ B /Ce, which is larger than the value expected for a Ce 3+ (refs 59 , 60 )). For the Yb-filled phases, P e ff =1.56, 2.76 and 2.71 μ B /Yb for Yb 0.9 Co 4 Sb 10.2 Sn 1.8 , Yb 0.9 Rh 4 Sb 10.2 Sn 1.8 and Yb 0.9 Ir 4 Sb 10.2 Sn 1.8 , respectively. For all three samples, the fits to Curie Weiss laws in the low-temperature regions yield effective moments that appear to be intermediate between those for Yb 3+ ( P eff =4.54 μ B /Yb for the free ion) and non-magnetic Yb 2+ ( P eff =0), however, due to the small energy differences between ground state and excited state electron configurations in Yb compounds, fits to the Curie Weiss law often do not reflect the true magnetic state of the system. Depressed values of effective moment for Yb have also been inferred from such fits for YbFe 4 Sb 12 ( P eff =3.09 μ B /Yb), for example ref. 61 . The new filled group 9 skutterudites that do not contain rare earths display temperature independent susceptibilities, with the exception of weak ‘Curie tails’ at low temperatures due to the presence of impurity spins. Almost all of the intrinsic susceptibilities are in fact diamagnetic for these materials, indicating that they are dominated by core diamagnetism, as expected from the electron-precise formulas. The magnetic susceptibilities at 150 K for the non-magnetic samples, also presented in Table 2 , are between −0.001 and −0.01 emu (mol formula unit) −1 . This indicates that the compounds do not display local moment behaviour, but rather band behaviour, even for the Co variants. It is of interest that the Co variants all display susceptibilities where no local moments are observed, as Co can be magnetic in many of its compounds. The implication is that the Co 3+ is in a low spin state, consistent with the chemical picture for these compounds, which has the t 2 g levels filled and the e g levels empty. More detailed study of the magnetic properties of the group 9 filled skutterudites will be of future interest. A 96 valence electron rule for stability of filled skutterudites is strongly supported by the current results and is analogous to the powerful 18 electron rule for half Heusler compounds. Using this counting rule, we have shown the existence of a very large new family of filled skutterudites based on the group 9 skutterudites CoSb 3 , RhSb 3 and IrSb 3 , stabilized by X site substitution to yield compounds with electron-precise formulas. The compounds were found through a combination of experimental studies and theoretical first principle calculations. In this work, 63 new filled skutterudite compositions based on the group 9 metals are reported, but by simple extension, for example, to the full 14 member rare-earth family, and to phosphides and arsenides in addition to the antimonides, we expect that several hundred new group 9-based filled skutterudite compounds can be found and characterized based on the concept presented here. This greatly expands the family of known filled skutterudites, an important solid structural family. The properties of the rare-earth-based filled skutterudites in other chemical families have proven to be very interesting especially for compounds based on the beginning (that is, Ce and Pr) and end (that is, Yb) of the magnetic rare-earth series. Those properties are strongly dependent on the spacing between rare earths, modified by varying the size of the X atoms, and also on the hybridization of the rare-earth orbitals with those of the transition metals present. The same effects are very likely to be exposed in the new skutterudite family described here through detailed study; their different transition metals in particular add a new degree of freedom by which the magnetic properties can be manipulated. Further, filled skutterudites with electron counts different from the electron-precise values have been made based on group 8 elements. In these cases, surprising properties like superconductivity can sometimes occur, for example, in LaRu 4 P 12 (ref. 62 ). The same kind of interesting electronic properties are also likely in our group 9 series with the correct combination of electron count and elemental constituents. Finally, the general approach employed here—to search for stable solid compounds of interesting transition element ions, even complex ones, by aiming at electron-precise (that is, Zintl) formulas—is likely to be a fruitful approach for expanding other families of solid compounds in the future. Calculation The electronic band structure calculations were performed in the framework of DFT using the WIEN2k [54] code with a full-potential linearized augmented plane-wave and local orbitals basis together with the Perdew Burke Ernzerhof parameterization [55] of the GGA as the exchange–correlation functional. In one case (see text), the MBJ [63] functional was also used (see Supplementary Fig. 1 ) The plane wave cutoff parameter RK MAX was set to 7 and the Brillouin zone was sampled by 500 k -points. To simulate the substitution of Sb by Sn, the virtual crystal approximation [64] , [65] was employed. The COHP [66] were generated by TB-LMTO atomic-sphere approximation (ASA) calculations using the Stuttgart code [65] . Exchange and correlation were treated by the local density approximation [67] . In the ASA method, space is filled with overlapping Wigner–Seitz (WS) spheres. The empty spheres were necessary in the calculation, and the WS sphere overlap was limited to no >16%. The basis set for the calculations included La (6 s , 6 p , 5 d and 4 f ), Co (4 s , 4 p and 3 d )/Rh (5 s , 5 p and 4 d )/Ir (6 s , 6 p and 5 d ) and Sb (5 s and 5 p ) wavefunctions. The convergence criterion was set to 10 − eV. A mesh of 6 × 6 × 6 k -points in the irreducible wedge of the first Brillouin zone was used to obtain all values. Experimental lattice constants were used and the free internal parameters were optimized by minimizing the forces. Synthesis and experiment Single-phase polycrystalline samples were synthesized from starting compositions A [Co/Rh/Ir] 4 Sb 11 Sn for A 1+ ions ( A =Li, Na and K), A [Co/Rh/Ir] 4 Sb 10 Sn 2 for A 2+ ions ( A =Ca, Sr and Ba) and A 0.9 [Co/Rh/Ir] 4 Sb 10.2 Sn 1.8 for A 3+ ions ( A =Ln=La, Ce, Pr, Gd and Yb). (Due to the large number of compounds described here, the formulas for the groups are abbreviated by the use of the square brackets for the group 9 element—in each case, pure Co, pure Rh and pure Ir variants were made.) The single-phase compositions reported here were determined in all cases by performing a series of systematic syntheses in extensive phase equilibria studies. The use of phase equilibria studies facilitated by powder XRD is a powerful, common method for determining the compositions of solids. The single-phase compositions reported here are those that yielded filled skutterudite compounds with y closest to 1 in A y B 4 X 12 . Samples were prepared by a solid-state reaction method. The alkali- and alkaline-earth-based groups are single phase for starting compositions at the ideal Zintl electron count, but for the lanthanide-antimony-based compounds, a more complex formula, with electrons in excess of the electron-precise count, was needed to make single-phase materials under our conditions. For A 1+ [Co/Rh/Ir] 4 Sb 11 Sn and A 2+ [Co/Rh/Ir] 4 Sb 10 Sn 2 , stoichiometric quantities of high-purity elemental Li/Na/K (99.999%), Ca/Sr/Ba (99.9%), Co (99.8%), Rh (99.99%) or Ir (99.99%), Sb (99.999%) and Sn (99.8%) were mixed, pressed into a pellet, put into an alumina crucible and then sealed in clean evacuated silica ampoules. The ampoules were slowly heated up to 600 °C and held for 10 h, then slowly heated up to 700 °C and held for 10 h. Then, they were removed from the furnace, thoroughly ground into powder, repressed into pellets and reheated at 700 °C for 10 h. This process was repeated two to four times until single-phase material was obtained. All the alkali- and alkaline-earth metals samples were made in two steps. For the first step, we mixed and ground the Co/Rh/Ir and Sb and Sn powders, and then put half the mixed powder in the bottom of the pellet die (in a glove box). The small pieces of alkali or alkaline-earth metals were then added into the middle, and the other half of the mixed power was put on the top, sandwiching the alkali/alkaline earth. The pellet was then pressed and put into a silica glass tube and heated to 600 °C at a rate of 1 °C min −1 for 10 h. Then, we opened the tube in a glove box and reground and repelletized the sample and reheated at 700 °C for 10 h. Critically, especially for the case of alkali filling of the skutterudite cavities, where a naive view might speculate that volatility or tube reaction might disrupt the synthesis, the internal surfaces of the silica ampoules were completely clean after the syntheses, showing no sign of attack or mass loss during the synthetic procedure. All the mixing and grinding processes were performed in a glove box ( P O2 and P H2O <1 p.p.m.). For comparison purposes, the binary skutterudites CoSb 3 , RhSb 3 and IrSb 3 were prepared by the same method. For Ln 0.9 [Co/Rh/Ir] 4 Sb 10.2 Sn 1.8 (Ln=La, Ce, Pr, Gd and Yb), precursor LnSn binaries or Ln[Co/Rh/Ir]Sn ternaries were first made by arc melting the elements. The as-prepared binaries and ternaries were then ground into powder and mixed with the appropriate stoichiometric quantities of high-purity elemental Co (99.8%), Rh (99.99%), Ir (99.99%), Sb (99.999%) and Sn (99.8%) powder, and heated as described above. Compounds based on phosphorous as the most electronegative element were also made, but for the rare-earth family only; Si or Ge were partially substituted for P to yield the Zintl electron count. For Ln[Co/Rh/Ir] 4 P 12− x [Ge/Si] x , (Ln=La, Ce, Pr and Nd), the precursor binaries or Ln[Co/Rh/Ir] 4 [Ge/Si] x ternaries were first made by arc melting the elements. Weight loss in this process was <1%. The as-prepared binaries or ternaries were then ground into powder and mixed with the appropriate stoichiometric quantities of elemental red P (99.9%), pressed into pellets and then sealed in clean evacuated silica ampoules. These ampoules were slowly heated to 400 °C, held for 10 h, and then slowly heated to 700 °C and held for 10 h; they were then slowly heated to 900 °C and held overnight. Finally, they were thoroughly ground into a powder, repressed into pellets, and reheated at 900 °C and held there overnight. Structural determination and physical properties The single-phase compositions determined in the phase equilibria studies were specified by powder XRD using a Bruker D8 Focus diffractometre with Cu Kα radiation and a graphite diffracted beam monochromator. The initial structural model for the structures that were quantitatively refined from the powder diffraction data was taken from that of LaRu 4 Sb 12 (ref. 68 ). The FullProf software suite was used for the Rietveld refinements. Peak shapes were modelled with the Thompson–Cox–Hastings pseudo–Voight profile convoluted with axial divergence asymmetry. The background was modelled with a Chebychev polynomial. The structures were refined in space group Im QUOTE with Co, Rh or Ir in the 8c sites and Sb/Sn in the 24g sites. The position of the A site ion was dependent on the specific compound, as described. In the final structural models, the structural parameters refined were the two positional coordinates ( x and y ) of the X atoms in position 24g, and when necessary, the position of the atom on the A atom site along the <111> direction and a small per cent of site mixing of A from the 2a onto the 8c site; all other structural parameters are fixed by symmetry. The formulas observed in the refinements were all consistent with the compositions determined from the phase equilibria studies. Similarly, the compositions of representative compounds tested by EDX were consistent with those compositions. Measurements of the temperature dependence of the electrical resistivity and magnetization were performed in a Quantum Design Physical Property Measurement System (PPMS) from 2 to 300 K. How to cite this article: Luo, H. et al . A large family of filled skutterudites stabilized by electron count. Nat. Commun. 6:6489 doi: 10.1038/ncomms7489 (2015).